Catalytic enantioselective oxidative coupling of saturated ethers with carboxylic acid derivatives Catalytic enantioselective C–C bond forming process through cross-dehydrogenative coupling represents a promising synthetic strategy, but it remains a long-standing challenge in chemistry. Here, we report a formal catalytic enantioselective cross-dehydrogenative coupling of saturated ethers with diverse carboxylic acid derivatives involving an initial oxidative acetal formation, followed by nickel(II)-catalyzed asymmetric alkylation. The one-pot, general, and modular method exhibits wide compatibility of a broad range of saturated ethers not only including prevalent tetrahydrofuran and tetrahydropyran, but also including medium- and large-sized cyclic moieties and acyclic ones with excellent enantioselectivity and functional group tolerance. The application in the rapid preparation of biologically active molecules that are difficult to access with existing methods is also demonstrated. The cross-dehydrogenative coupling (CDC) of two readily available C–H components has emerged as a powerful approach for C–C bond construction whereby the only loss is H 2 formally [1] , [2] , [3] . The design of the catalytic asymmetric variant is particularly attractive, but remains a challenging task [4] , [5] , [6] . Although impressive progress has been made in enantioselective CDC during the last decade, current studies predominantly focused on N -arylated amine [7] , [8] , [9] , [10] , [11] , [12] , [13] , [14] , [15] , [16] , [17] , [18] , [19] and xanthese substrates [20] , [21] , [22] , [23] , [24] , [25] . In contrast, enantioselective CDC of ethers has remained scarce, and the unique existing two examples still focused on specific, activated benzylic and allylic ethers [26] , [27] . Our group described an enantioselective bimolecular CDC of cyclic benzylic ethers and aldehydes with high enantioselectivity [26] . Scheidt reported a delicate asymmetric intramolecular CDC of allylic ethers with appended β-keto esters, providing substituted tetrahydropyran-4-ones with excellent diastereo- and enantioselectivities [27] . On the other hand, optically pure saturated ethers with diverse α-alkyl substitutions represent ubiquitous structural motifs in numerous bioactive natural products and synthetic pharmaceuticals [28] , [29] , [30] . However, each catalytic asymmetric method is typically suitable for a single class of tetrahydrofuran (THF), tetrahydropyran (THP), or acyclic ether skeleton with a specific α-alkyl substitution pattern [31] , [32] , [33] , [34] , [35] , [36] , [37] , [38] , [39] , [40] , [41] , [42] , [43] , [44] , [45] , [46] . A general and modular catalytic enantioselective method to rapidly access saturated ethers with diverse skeletons and α-alkyl substituent patterns from readily available starting materials has remained elusive. Diverse saturated ether skeletons are basic feedstocks, and many of which, such as THF, THP, and diethyl ether, are daily used solvents in both academia and industry. Therefore, the development of catalytic asymmetric synthetic method starting from such abundant, low value chemical resources and sp 3 C–H components is highly desirable. Herein, we report a formal catalytic enantioselective CDC of saturated ethers and carboxylic acid derivatives. The one-pot method exhibits wide compatibility of a broad range of saturated cyclic and acyclic ethers with excellent enantioselectivity. The application in the rapid preparation of biologically active molecules that are difficult to access with existing methods has also been demonstrated. Reaction design Presumably, two major challenges hamper the design of catalytic asymmetric oxidative coupling starting from saturated ethers. First, due to the low reactivity of saturated ethers, the C–H cleavage process requires strongly oxidative conditions, making the compatibility with delicate asymmetric catalysis system difficult to achieve [47] . Second, while catalytic asymmetric addition to aromatic oxocarbenium ions has received considerable attentions [48] , [49] , [50] , [51] , [52] , [53] , the lack of any site on non-aromatic oxocarbenium ions for substrate–catalyst interactions makes asymmetric synthesis of α-substituted saturated ethers via such intermediates remains elusive [54] , [55] , [56] . Herein, we communicate a one-pot catalytic asymmetric synthetic method involving a broad range of saturated ethers and diverse carboxylic acid derivatives as starting materials. The one-pot synthetic method was designed as follow: saturated ether reacting with a combination of a protic additive and peroxide furnished a racemic acetal, which then ionized to corresponding oxocarbenium intermediate for enantioselective C–C bond forging process. 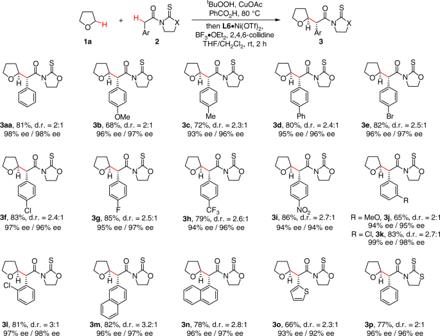Fig. 1 The scope of α-aryl acetic acid derivatives. Conditions: PhCOOH (0.5 mmol, 2.5 equiv), CuOAc (2.5 mol%),tBuOOH in decane (2.5 equiv) in THF (1.0 mL) at 80 °C for 2 h, followed by 2 (1.0 equiv), L6·Ni(OTf)2(10 mol%), 2,4,6-collidine (3.0 equiv) and BF3·OEt2(4.0 equiv) in THF/CH2Cl2(0.3 mL/0.1 mL) at rt for 2 h Reaction condition optimization The reaction of THF ( 1a ) and acetyloxazolidinone 2a was selected for optimization using bisoxazoline L1 /Mg(ClO 4 ) 2 as chiral catalyst (Table 1 ) [57] , [58] , [59] , [60] , [61] . An initial survey revealed that oxidation of THF with hexanoic acid proceeded smoothly in the presence of t BuOOH and a suitable additive, including TBAI, Fe(acac) 3 , Cu(acac) 2 , Cu(OAc) 2 , and CuOAc [62] . However, these catalytic amount of additive exhibited a dramatic effect on the subsequent enantioselective C–C bond forming reaction in the presence of BF 3 ·OEt 2 /2,4,6-collidine, and CuOAc was identified to be optimal, providing expected 3a in 14% yield with 17% ee as a separable mixture of diastereomers (d.r. = 50:50) (entries 1–5, Table 1 ). Lowing the loading of CuOAc afforded an improved reaction efficiency and ee (entry 6, Table 1 ). Acetyloxazolidinethione 2aa proved to be a better component with regard to ee and yield (entry 7, Table 1 ). An extensive investigation of the combination of Lewis acid with chiral ligands L1 - L6 revealed that diphosphine L6 and Ni(OTf) 2 provided the highest yields and enantiocontrol (entries 8–17, Table 1 ). By using pre-prepared L6 ·Ni(OTf) 2 as catalyst, the yield increased from 55% to 61% without detriment to ee (entry 18, Table 1 ). By increasing the loading of BF 3 ·OEt 2 , the enantioselectivity and yield were improved to 90% and 86%, respectively (entry 19, Table 1 ). The reaction was also highly dependent on the solvent choice, and the nucleophilic addition stage worked the best in a mixed THF/CH 2 Cl 2 (entry 20, Table 1 ). The effect of protic additives was further explored, and reaction with PhCOOH furnished the product in 81% yield and 98% ee as a 67:33 mixture of diastereomers, which were separable through silica gel chromatography (entry 21, Table 1 ). The combination of BF 3 ·OEt 2 /2,4,6-collidine proved to be crucial to the expected reactivity (See Supplementary Table 1 ). No desired product was detected when BF 3 ·OEt 2 was replaced with TMSOTf or 2,4,6-collidine with diisopropylethylamine. Lowering the reaction temperature for the asymmetric C–C bond forming process did not provide any improvement on the diastereoselectivity (entry 22, Table 1 ). Table 1 Reaction condition optimization a Full size table Scope of acetic acid derivatives The scope of acetic acid derivatives was then explored (Fig. 1 ). A variety of electron-donating and -withdrawing substituents at the ortho -, meta -, and para -positions of the aryl ring were well compatible with the reaction conditions, providing respective α-aryl acetamide substituted THF 3a – 3l in good yields with moderate diastereoselectivity and excellent enantioselectivity (93–98% ee) for both isomers. (α-Heteroaryl) 3o , as well as (α-nathphyl)acyl oxazolidinethiones 3m and 3n were suitable components in high enantioselectivities. N -phenylacyl thiazolidinethione was also well tolerated, as demonstrated by the generation of 3p in 96% ee. Fig. 1 The scope of α-aryl acetic acid derivatives. Conditions: PhCOOH (0.5 mmol, 2.5 equiv), CuOAc (2.5 mol%), t BuOOH in decane (2.5 equiv) in THF (1.0 mL) at 80 °C for 2 h, followed by 2 (1.0 equiv), L6·Ni(OTf) 2 (10 mol%), 2,4,6-collidine (3.0 equiv) and BF 3 ·OEt 2 (4.0 equiv) in THF/CH 2 Cl 2 (0.3 mL/0.1 mL) at rt for 2 h Full size image To further expand the synthetic utility of the method, we next investigated the possibility of α-alkenyl acetic acid derivatives as coupling components (Fig. 2 ). Thiazolidinethione 3r was superior to oxazolidinethione 3q in terms of ee and yield. In general, the reaction exhibited excellent regioselectivity, and the alkylation occurred exclusively at the α-position of 3-butenoyl derivatives with olefin geometry highly conserved. Electronically varied γ-aryl substituted 3-butenoyl 2s and 2t together with γ-alkyl substituted 2u – 2x were competent components, providing corresponding 3s – 3w in good yields with 90–96% ee. γ-Disubstituted 2y and 2z were also well tolerated in excellent enantiocontrol. The method had an excellent functional group tolerance, with common functionalities including terminal alkyne ( 3ba ), benzoate ( 3bb ), silyl ether ( 3bc ), halide ( 3bd ), and azide ( 3be ) well tolerated in 90–92% ee for further manipulation. No expected product 3bf was observed when α-alkyl acetic acid derivative 2bf was used as the coupling partner. Fig. 2 The scope of α-alkenyl acetic acid derivatives. Conditions: PhCOOH (0.5 mmol, 2.5 equiv), CuOAc (2.5 mol%), t BuOOH in decane (2.5 equiv) in THF (1.0 mL) at 80 °C for 2 h, followed by 2 (1.0 equiv), L5·Ni(OTf) 2 (10 mol%), 2,4,6-collidine (3.0 equiv), and BF 3 ·OEt 2 (4.0 equiv) in CH 3 CO 2 CH 3 /CH 2 Cl 2 (0.3 mL/0.1 mL) at rt for 2 h Full size image Scope of saturated ethers The scope of saturated cyclic ethers was next examined (Fig. 3 ). Under the standard conditions, 1,1-disubstituted THF proved to be competent substrates, furnishing trisubstituted THF 4a – 4c in good yields with 94–96% ee and moderate d.r.. Enantioselective reaction of THP with α-aryl and α-vinyl substituted acetic acid derivatives also proceeded smoothly, giving corresponding 4d – 4j with excellent enantiocontrol. The success in the prevalent THF and THP frameworks encouraged us to further investigate the feasibility of enantioselective functionalization of larger cyclic ethers. Delightedly, medium-sized cyclic, aliphatic ethers, such as oxepane and oxocane, were tolerated, providing 4k and 4l in 96% ee and 92% ee, respectively. Albeit slightly decreased efficiency, large-sized cyclic, saturated ethers were also identified as competent substrates, as demonstrated by the generation of 13-membered 4m and 16-membered 4n in 96% ee and 95% ee. Although the scope of saturated cyclic ethers was not exclusively investigated, these results provide a proof-of-concept for the generality and modularity of the asymmetric synthetic method. Fig. 3 The scope of cyclic saturated ethers. Conditions: PhCOOH (0.5 mmol, 2.5 equiv), CuOAc (2.5 mol%), t BuOOH in decane (3.0 equiv) in ether (1.0 mL) at 80 °C for 6–12 h, followed by 2 (1.0 equiv), L5·Ni(OTf) 2 or L6·Ni(OTf) 2 (10 mol%), 2,4,6-collidine (3.0 equiv), and BF 3 ·OEt 2 (4.0 equiv) in CH 2 Cl 2 (0.4 mL) at rt for 2 h Full size image The tolerance of large-sized, cyclic ether prompted us to further explore the generality of the method for acyclic saturated ethers (Fig. 4 ). Pleasingly, enantioselective reaction of commonly used solvents, such as diethyl ether, dipropyl ether, and dibutyl ether, with 2aa proceeded smoothly, providing 6a – 6c in good yields with 90–94% ee. Aside from symmetric acyclic ethers, unsymmetric ones also proved to be suitable substrates, as demonstrated by the highly enantioselective reaction of methyl n-butyl ether ( 6d ) and methyl n-hexyl ether ( 6e ). The reaction exhibited excellent regioselectivity, and no substitution at primary C–H bond was observed. Acyclic ethers bearing a variety of commonly encountered functional groups, such as ether ( 6f ), halide ( 6g ), and acetate ( 6h ), were also well tolerated for further manipulation. No improvement on the diastereoselectivity was observed when bulky tert -butyl ethyl ether ( 6i ) was employed. Fig. 4 The scope of acyclic saturated ethers. Conditions: PhCOOH (0.5 mmol, 2.5 equiv), CuOAc (2.5 mol%), t BuOOH in decane (3.0 equiv) in ether (1.0 mL) at 80 °C for 6–12 h, followed by 2 (1.0 equiv), L6·Ni(OTf) 2 (10 mol%), 2,4,6-collidine (3.0 equiv), and BF 3 ·OEt 2 (4.0 equiv) in CH 2 Cl 2 (0.4 mL) at rt for 2 h Full size image Synthetic applications The synthetic utilities of the method was next explored (Fig. 5 ). First, the oxa- and thiazolidinethione moieties can be readily converted to other synthetically valuable functional groups. For example, the adduct 3a was converted to corresponding alcohol 7 , ester 8 , thioester 9 , and Weinreb amide 10 in high efficiency with the ee highly conserved (Fig. 5a ). Enantiopure diastereomers 12a and 12b are potent and selective dopamine transporter inhibitors (Fig. 5b ) [63] . However, traditional synthetic method, which relied on menthol or 1-indanol mediated resolution technology, required seven steps for each isomer preparation starting from 3,4-dihydro-2 H -pyran. Our method exhibited moderate diastereoselectivity, which afforded an opportunity to rapidly access both 12a and 12b in excellent ee through a two-step process consisting of asymmetric reaction of THP ( 1d ) with 11 and esterification. 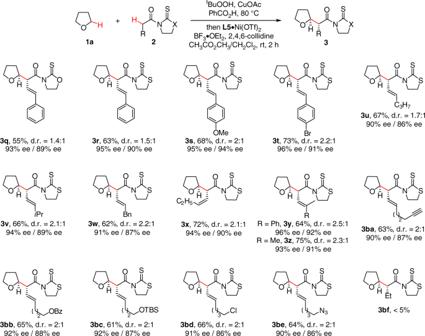Fig. 2 The scope of α-alkenyl acetic acid derivatives. Conditions: PhCOOH (0.5 mmol, 2.5 equiv), CuOAc (2.5 mol%),tBuOOH in decane (2.5 equiv) in THF (1.0 mL) at 80 °C for 2 h, followed by 2 (1.0 equiv), L5·Ni(OTf)2(10 mol%), 2,4,6-collidine (3.0 equiv), and BF3·OEt2(4.0 equiv) in CH3CO2CH3/CH2Cl2(0.3 mL/0.1 mL) at rt for 2 h Second, given the tolerance of a broad range of carboxylic acid derivatives, we envisioned that removing the exocyclic stereocenter would further enhance the synthetic utility of the protocol. Therefore, we designed a concise two-step sequence involving DIBAL-H mediated reduction of oxa- or thiazolidinethione to aldehyde followed by Ru(PPh 3 ) 3 Cl catalyzed decarbonylation, providing α-alkyl substituted saturated ethers 13 – 17 that are difficult to prepare by other methods (Fig. 5c ). Fig. 5 Synthetic utilities. a Transformations of oxa- and thiazolidinethiones to other synthetically valuable functional groups. b Rapid synthesis of two dopamine transporter inhibitors. c Removal of the oxa- and thiazolidinethione moieties Full size image Control experiments were conducted to gain a preliminary understanding of the reaction mechanism (Fig. 6 ). First, in the presence of CuOAc and t BuOOH, THF ( 1a ) reacted with PhCO 2 H giving acetate 18 in 88% yield (Fig. 6a ). Subjecting 18 to the standard condition furnished expected 3aa with comparable results to that observed in the reaction starting from THF ( 1a ) (Fig. 6b ). The observations implied the intermediacy of 18 in the process. Second, the alkylation of 18 with 2aa proceeded smoothly under the standard reaction condition in the absence of oxidation elements (Fig. 6c ). No expected 3aa was observed when the combination of L6 and CuOAc was used as the catalyst (Fig. 6d ). These results suggested that the species binding to diphosphine ligand should be Ni(OTf) 2 but not CuOAc. Fig. 6 Mechanistic studies. a Reaction intermediate identification. b Asymmetric coupling of 18 with 2aa. c Asymmetric coupling of 18 with 2aa in the absence of CuOAc. d Identification of the real metal catalyst for the asymmetric coupling Full size image Based on the above observations, a plausible catalytic cycle is outlined in Fig. 7 . Carboxylic acid derivative 2aa coordinates with L6 ·Ni(OTf) 2 complex giving rise to 19 , in which the acidity of the hydrogen α to the carbonyl moiety increases. 2,4,6-Collidine promotes the enolization of 19 providing chiral Ni-bound Z -enolate 20 [64] . 20 Reacts with cyclic oxocarbenium 21 generated in situ from acetal 18 and BF 3 ·OEt 2 yielding 22 . Product dissociation completes the catalytic cycle. Notably, no reactivity was detected when diisopropylethylamine was used instead of 2,4,6-collidine, indicating that the role of latter might not simply act as a base. Fujioka and Kita reported that in the presence of a suitable Lewis acid, the acetal reacted with 2,4,6-collidine furnishing corresponding pyridinium-type salt [65] . During our in situ 1 H NMR study of the mixture of acetal 18 , BF 3 ·OEt 2 , and 2,4,6-collidine, a peak at δ ~ 6.4 ppm was observed, which is characteristic for such type of pyridinium species [65] , [66] . Accordingly, we envisioned that 2,4,6-collidine might react with oxocarbenium 21 reversibly furnishing pyridinium 23 . Adduct 23 possessing weak electrophilicity might be considered as a reservoir of 21 to prevent the decomposition before the capture by enolate 20 . 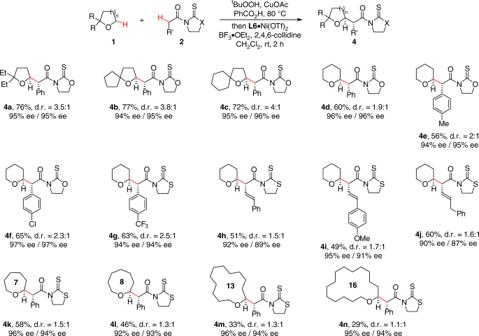Fig. 3 The scope of cyclic saturated ethers. Conditions: PhCOOH (0.5 mmol, 2.5 equiv), CuOAc (2.5 mol%),tBuOOH in decane (3.0 equiv) in ether (1.0 mL) at 80 °C for 6–12 h, followed by 2 (1.0 equiv), L5·Ni(OTf)2or L6·Ni(OTf)2(10 mol%), 2,4,6-collidine (3.0 equiv), and BF3·OEt2(4.0 equiv) in CH2Cl2(0.4 mL) at rt for 2 h Fig. 7 A proposed catalytic cycle. The possible reaction pathway based on our studies and previous literature Full size image The stereochemical induction model based on the Ni-bound Z -enolate with chiral bidentate phosphine ligand L6 (MeO-BIPHEP) was proposed in Fig. 8 . The P -bound phenyl group on the ligand (in red) shields the top face ( Re face) of the enolate substrate (in blue), which disfavors the electrophilic attack by the oxocarbenium intermediate. In contrast, the addition of the oxocarbenium ion to the Si face of the enolate substrate is favored due to less repulsive interactions with the ligand. This model is consistent with the experimentally observed stereochemistry. The low to moderate diastereoselectivity observed for saturated ethers might be ascribed to the lack of Lewis basic site on corresponding oxocarbenium ion intermediates for substrate–catalyst interactions. Fig. 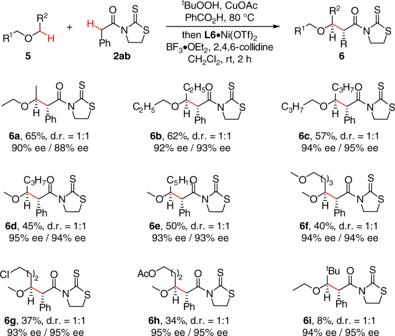Fig. 4 The scope of acyclic saturated ethers. Conditions: PhCOOH (0.5 mmol, 2.5 equiv), CuOAc (2.5 mol%),tBuOOH in decane (3.0 equiv) in ether (1.0 mL) at 80 °C for 6–12 h, followed by 2 (1.0 equiv), L6·Ni(OTf)2(10 mol%), 2,4,6-collidine (3.0 equiv), and BF3·OEt2(4.0 equiv) in CH2Cl2(0.4 mL) at rt for 2 h 8 Stereochemical induction model with chiral Ni-bound Z -enolate. The geometry was optimized at the B3LYP/LANL2DZ–6–31G(d) level Full size image In summary, a one-pot catalytic enantioselective reaction of saturated ethers with diverse carboxylic acid derivatives is described. The general and modular method exhibits wide compatibility of a broad range of saturated cyclic ethers not only including prevalent THF and THP, but also including medium- and large-sized cyclic moieties with excellent enantioselectivity and functional group tolerance. The generality of the method is further demonstrated by application in saturated acyclic ethers. The synthetic application in the rapid preparation of biologically active molecules that are difficult to access with existing methods is demonstrated. We envision that the general, modular, and highly enantioselective reaction of abundant, low value saturated ethers outlined herein will provide a topologically straightforward synthetic planning for both complex target molecules and a plethora of analogs for lead discovery and optimization. 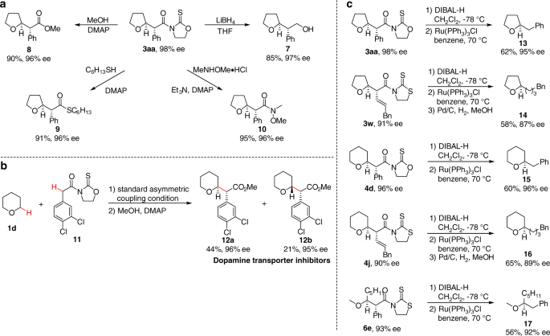Fig. 5 Synthetic utilities.aTransformations of oxa- and thiazolidinethiones to other synthetically valuable functional groups.bRapid synthesis of two dopamine transporter inhibitors.cRemoval of the oxa- and thiazolidinethione moieties 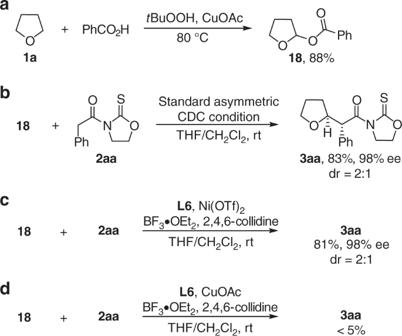Fig. 6 Mechanistic studies.aReaction intermediate identification.bAsymmetric coupling of 18 with 2aa.cAsymmetric coupling of 18 with 2aa in the absence of CuOAc.dIdentification of the real metal catalyst for the asymmetric coupling General procedure for the reaction of THF (1a) with 2aa In an oven-dried Teflon septum screw-capped tube, PhCOOH (61 mg, 0.5 mmol), CuOAc (0.6 mg, 0.005 mmol, 2.5 mol%), and t BuOOH in decane (0.5 mmol) were added to THF (1.0 mL). 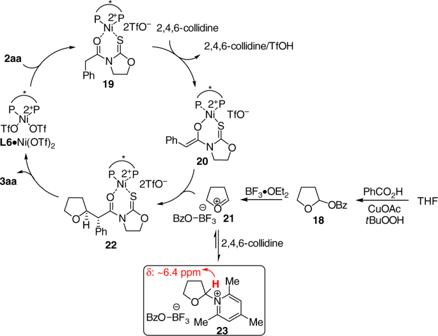Fig. 7 A proposed catalytic cycle. The possible reaction pathway based on our studies and previous literature 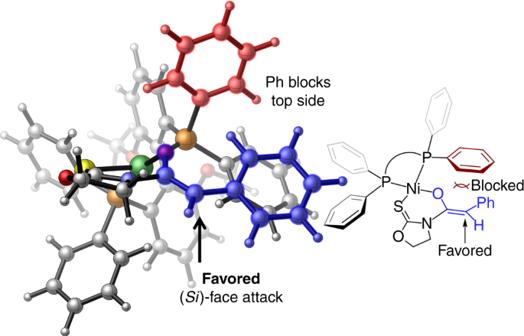Fig. 8 Stereochemical induction model with chiral Ni-boundZ-enolate. The geometry was optimized at the B3LYP/LANL2DZ–6–31G(d) level The solution was stirred at 80 °C for 2 h before the solvent was evaporated. Then carboxylic acid derivative 2aa (44.3 mg, 0.2 mmol), L6· Ni(OTf) 2 (18.7 mg, 0.02 mmol), 2,4,6-collidine (79.3 μL, 0.6 mmol), and BF 3 ·OEt 2 (98.7 μL, 0.8 mmol) in THF/CH 2 Cl 2 (0.3 mL/0.1 mL, v-v) was added. After stirring at rt for 2 h, solvents were removed and the residue was purified by silica gel column chromatography (CH 2 Cl 2 /ethyl acetate = 99:1) giving the expected 3aa in 81% yield (47.2 mg) with 98% ee as a separable mixture of diastereomers (d.r. = 2:1).